Towards intrinsic charge transport in monolayer molybdenum disulfide by defect and interface engineering Molybdenum disulfide is considered as one of the most promising two-dimensional semiconductors for electronic and optoelectronic device applications. So far, the charge transport in monolayer molybdenum disulfide is dominated by extrinsic factors such as charged impurities, structural defects and traps, leading to much lower mobility than the intrinsic limit. Here we develop a facile low-temperature thiol chemistry route to repair the sulfur vacancies and improve the interface, resulting in significant reduction of the charged impurities and traps. High mobility >80 cm 2 V −1 s −1 is achieved in backgated monolayer molybdenum disulfide field-effect transistors at room temperature. Furthermore, we develop a theoretical model to quantitatively extract the key microscopic quantities that control the transistor performances, including the density of charged impurities, short-range defects and traps. Our combined experimental and theoretical study provides a clear path towards intrinsic charge transport in two-dimensional dichalcogenides for future high-performance device applications. Despite its great promise as a two-dimensional (2D) channel material for logic transistors [1] , [2] , integrated circuits [3] , [4] and photodetectors [5] , [6] , the charge transport in monolayer of molybdenum disulfide (MoS 2 ) is still far away from the intrinsic limit. Theoretically, the phonon-limited mobility is ~410 cm 2 V −1 s −1 at room temperature and is weakly dependent on carrier density until ~10 13 cm −2 , where electron–electron scattering starts to play important roles [7] . Experimentally, however, very different behaviour is observed regardless of the sample preparation method. First, the electron mobility in backgated monolayer MoS 2 devices is limited to ~40 cm 2 V −1 s −1 at room temperature, an order of magnitude lower than the phonon limit [2] , [8] , [9] , [10] . Second, the mobility is found to increase with carrier density even beyond 10 13 cm −2 (refs 2 , 9 ). Third, at low carrier density, the charge transport is dominated by hopping mechanism [11] , [12] . Fourth, a metal–insulator transition (MIT) is observed at high carrier densities on the order of 10 13 cm −2 , but the underlying mechanism remains debated [2] , [8] , [9] . These observations clearly point to the existence of extrinsic factors that dominate charge transport in monolayer MoS 2 . Charged impurities (CI) [2] , [13] , short-range defects [11] and localized states [11] , [14] , [15] , among others, are believed to strongly influence electron transport. However, a comprehensive physical picture that explains all of above-mentioned transport phenomena and provides quantitative and microscopic insights into the impurities is still lacking. Owing to its atomic thickness, electrons in monolayer MoS 2 are more susceptible to impurities both inside MoS 2 and at the dielectric interface. Therefore, the engineering of defects and interface represents a logical route to further improve MoS 2 device performance. Recently, the use of thiol-terminated SiO 2 (ref. 16 ), boron nitride [17] and suspended structure [18] were found to improve the mobility of monolayer MoS 2 devices by several folds, showing the importance of interface. However, their mobility values are still much lower than the intrinsic limit, indicating that other sources of impurities, most likely inside MoS 2 , are still present. In this work, we show that sulfur vacancies (SVs), which are the main type of intrinsic defects in MoS 2 (ref. 11 ), can be effectively repaired by (3-mercaptopropyl)trimethoxysilane (MPS) under mild annealing, resulting in significant reduction of CI and short-range scattering. Monolayer MoS 2 with both sides treated by MPS exhibits a record-high mobility of 81 cm 2 V −1 s −1 (320 cm 2 V −1 s −1 ) at room temperature (low temperature), much higher than untreated samples. In addition, we show that MIT in MoS 2 is due to localized trap states, which can be modulated by improving the sample and interface quality. A theoretical model that takes into account the major scattering sources (phonon, CI and short-range defects) and localized charge traps is developed to quantitatively understand the scaling of mobility, conductivity and MIT in monolayer MoS 2 . By fitting the experimental data, we are able to extract key microscopic quantities including the density of CI, short-range defects and charge traps, as well as derive a transport phase diagram for MoS 2 . The quantitative information also allows us to discuss the possible origins of these extrinsic factors, which serve as the basis for further device optimization. Repair of SVs by thiol chemistry The monolayer MoS 2 samples studied here are obtained by mechanical exfoliation from bulk crystals ( Supplementary Fig. 1 ). A high density of SV exists in as-exfoliated MoS 2 as demonstrated in earlier works [11] , [19] . These defects, which can act as catalytic sites for hydrodesulfurization reactions [20] , [21] , are chemically reactive. Therefore, it is possible to repair the SV by thiol chemistry. Here, we choose a specific molecule MPS ( Fig. 1 inset) for two reasons. (i) The S-C bond in MPS is weaker than other thiol molecules like dodecanethiol due to the acidic nature of CH 3 -O- groups, leading to a low energy barrier for the reaction [22] . (ii) The trimethoxysilane groups in MPS react with the SiO 2 substrate to form a self-assembled monolayer [23] (SAM, Supplementary Fig. 2 ). The SAM layer can effectively passivate the MoS 2 /SiO 2 interface, while the outstanding thiol group can also repair the SV on the bottom side of MoS 2 , which is otherwise difficult to access. This unique property of MPS allows us to systematically compare three types of MoS 2 samples: as-exfoliated on SiO 2 , top-side (TS) treated on SiO 2 and double-side (DS) treated. For the MPS treatment, we used a liquid-phase process [22] , followed by 350°C annealing in forming gas to repair the SV (see Methods and Supplementary Fig. 3 for details of sample preparation and characterization). 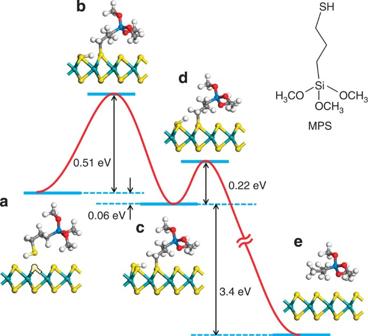Figure 1: Kinetics and transient states of the reaction between a single SV and MPS. There are two energy barriers, the first one (0.51 eV) is due to the S-H bond breaking, and the second one (0.22 eV) is due to S-C bond breaking. (a–e) Plots the initial, transient and final states of the reaction. The SV in the initial state is illustrated by dashed line in (a). The inset shows the chemical structure of MPS. Figure 1: Kinetics and transient states of the reaction between a single SV and MPS. There are two energy barriers, the first one (0.51 eV) is due to the S-H bond breaking, and the second one (0.22 eV) is due to S-C bond breaking. ( a – e ) Plots the initial, transient and final states of the reaction. The SV in the initial state is illustrated by dashed line in ( a ). The inset shows the chemical structure of MPS. Full size image We first study the reaction kinetics of SV and MPS by density functional theory ( Fig. 1 ). The reaction can be described by HS(CH 2 ) 3 Si(OCH 3 ) 3 +SV →CH 3 (CH 2 ) 2 Si(OCH 3 ) 3 ( Supplementary Fig. 4 ; Supplementary Movie 1 ), which is exothermic with the enthalpy change of −333.3 kJ mol −1 of MPS. The reaction process comprises two steps with an energy barrier of 0.51 eV and 0.22 eV, respectively. In the first step ( Supplementary Fig. 5 ), MPS chemically absorbs onto an SV through the sulfur atom, and then it cleaves the S-H bond and forms a thiolate surface intermediate. The dissociated H atom is bonded to a neighbouring S atom. The second step involves cleavage of the S-C bond and hydrogenation of the thiolate intermediate to form the final product trimethoxy(propyl)silane ( Supplementary Fig. 6 ). We note that the two-step process agrees well with earlier thiol absorption experiments on defective MoS 2 (refs 20 , 22 ). The relatively low energy barriers also facilitate the reaction to occur at low temperature. To quantify the effect of MPS treatment on sample quality, we perform aberration-corrected transmission electron microscopy (TEM) on as-exfoliated and TS-treated monolayer MoS 2 . 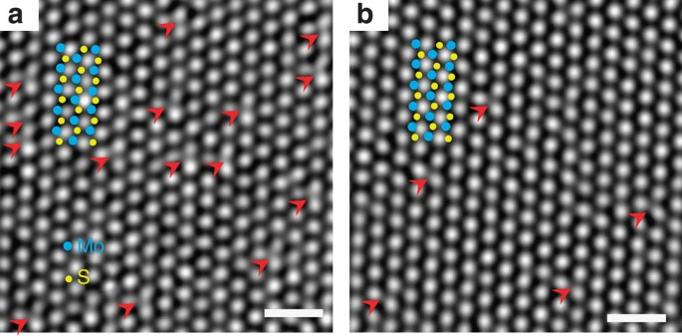Figure 2: High-resolution aberration-corrected TEM images. (a) As-exfoliated and (b) TS-treated monolayer MoS2sample, showing the significant reduction of SV by MPS treatment. The SVs are highlighted by red arrows. The overlaid blue and yellow symbols mark the position of Mo and S atoms, respectively. Scale bar, 1 nm. Detailed intensity profile analysis and histogram of SV density are shown inSupplementary Fig. 9. Figure 2 compares high-resolution TEM images of a typical as-exfoliated and TS-treated sample. The SVs can be clearly distinguished by analysing the intensity profile [11] as shown in Supplementary Fig. 9 . Statistical analysis (from more than 15 areas in each case) indicates that the density of SV is reduced from ~6.5 × 10 13 cm −2 for the as-exfoliated samples to ~1.6 × 10 13 cm −2 for the TS-treated samples ( Supplementary Fig. 9c,d ). Owing to the difficulty in making TEM samples, we are not able to characterize the DS-treated MoS 2 , where further reduction of SV is expected. During the course of TEM experiment, we have paid great attention to minimize the knock-on damage and lattice reconstruction caused by electron beam irradiation [24] by limiting the exposure time to <30s and the current density to below 10 6 e nm −2 S −1 (ref. 11 ). The SV generation rate induced by electron irradiation under our experimental conditions was very low, ~5.6 × 10 10 cm −2 S −1 (ref. 11 ). Therefore, the SVs in Fig. 2 are believed to be intrinsic rather than induced by electron irradiation. Figure 2: High-resolution aberration-corrected TEM images. ( a ) As-exfoliated and ( b ) TS-treated monolayer MoS 2 sample, showing the significant reduction of SV by MPS treatment. The SVs are highlighted by red arrows. The overlaid blue and yellow symbols mark the position of Mo and S atoms, respectively. Scale bar, 1 nm. Detailed intensity profile analysis and histogram of SV density are shown in Supplementary Fig. 9 . Full size image Electrical transport properties Next, we systematically investigated the effect of MPS treatment on electrical transport properties of MoS 2 . We fabricated backgated field-effect transistors (FETs) on as-exfoliated, TS-treated and DS-treated monolayer MoS 2 samples, and carried out electrical measurements in high vacuum with a standard four-probe technique, unless otherwise stated (see Methods for details of device fabrication and measurement). All the devices exhibited very small hysteresis at room temperature, which became even smaller as they were cooled down ( Supplementary Fig. 10 ). Therefore, in the following we only present electrical data from the forward sweep. 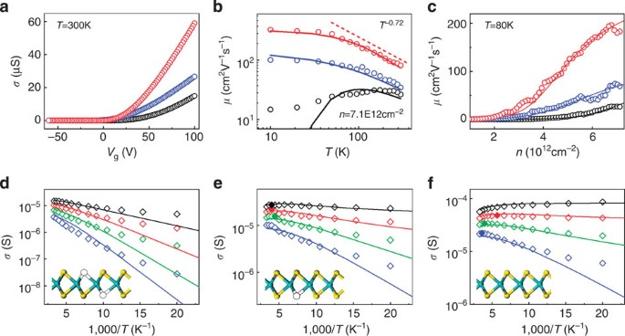Figure 3: The effect of defect and interface engineering on monolayer MoS2charge transport. (a) Typicalσ-Vgcharacteristics for as-exfoliated (black), TS-treated (blue) and DS-treated (red) monolayer MoS2atT=300 K. (b)μ-Tcharacteristics for the three devices atn=7.1 × 1012cm−2. Solid lines are the best theoretical fittings. The dashed red line showsT−0.72scaling. (c)μ-ncharacteristics for the three devices atT=80 K. Solid lines are the best theoretical fittings. (d–f) Arrhenius plot ofσ(symbols) and theoretical fittings (lines) for the as-exfoliated (d), TS-treated (e) and DS-treated (f) MoS2. From top to bottom,n=7.0, 6.0, 5.0 and 4.0 × 1012cm−2, respectively. The critical points of the MIT are highlighted by solid symbols in (e) and (f). Insets in (d–f) show the cartoon illustration of the corresponding MoS2samples undergone different treatments. Figure 3a shows the four-probe conductivity σ =( I ds )/(Δ V )( L )/( W ) as a function of backgate voltage V g for three representative devices at room temperature (300 K), where I ds is the source-drain current; Δ V , L and W are the voltage difference, distance and sample width between the two voltage probes, respectively. The MPS-treated samples show improved σ compared with the as-exfoliated one, indicating higher sample and interface quality. At carrier density n = C g V g =7.1 × 10 12 cm −2 ( C g =11.6 nF cm −2 is the gate capacitance for 300 nm SiO 2 dielectrics), the DS-treated sample shows σ =1.52 e 2 h −1 and field-effect mobility μ =(d σ )/( C g d V g ) =81 cm 2 V −1 s −1 . To our best knowledge, this is the highest room-temperature field-effect mobility reported so far for monolayer MoS 2 regardless of the device geometry [2] , [8] , [9] , [10] . Figure 3: The effect of defect and interface engineering on monolayer MoS 2 charge transport. ( a ) Typical σ - V g characteristics for as-exfoliated (black), TS-treated (blue) and DS-treated (red) monolayer MoS 2 at T =300 K. ( b ) μ - T characteristics for the three devices at n =7.1 × 10 12 cm −2 . Solid lines are the best theoretical fittings. The dashed red line shows T −0.72 scaling. ( c ) μ - n characteristics for the three devices at T =80 K. Solid lines are the best theoretical fittings. ( d – f ) Arrhenius plot of σ (symbols) and theoretical fittings (lines) for the as-exfoliated ( d ), TS-treated ( e ) and DS-treated ( f ) MoS 2 . From top to bottom, n =7.0, 6.0, 5.0 and 4.0 × 10 12 cm −2 , respectively. The critical points of the MIT are highlighted by solid symbols in ( e ) and ( f ). Insets in ( d – f ) show the cartoon illustration of the corresponding MoS 2 samples undergone different treatments. Full size image To gain further insights into the charge transport physics, we performed variable-temperature electrical measurements down to 10 K. Surprisingly, the three types of devices exhibit very different behaviour ( Fig. 3 ; Supplementary Fig. 11 ). For the as-exfoliated sample, σ monotonically decreases during cooling over the entire range of n , indicating an insulating behaviour ( Fig. 3d ; Supplementary Fig. 11a ). For the DS-treated sample, the transfer curves all intersect near V g =80 V (corresponding to n ~5.7 × 10 12 cm −2 , Supplementary Fig. 11c ), which is a signature of MIT. Metallic and insulating behaviours are observed down to the base temperature for n >6.6 × 10 12 cm −2 and n <3.5 × 10 12 cm −2 , respectively. At intermediate n , the σ-T characteristics are not monotonic, and MIT occurs within our experimental temperature range (solid symbols in Fig. 3f ). For the TS-treated sample, MIT is observed for n >4.7 × 10 12 cm −2 (solid symbols in Fig. 3e ), while insulating behaviour is always observed at low temperatures ( Fig. 3e ; Supplementary Fig. 11b ). As we shall see later, these distinct transport behaviours precisely reflect the quality of the MoS 2 and interface. The scaling behaviour of μ is also very different for the three samples ( Fig. 3b,c ). The as-exfoliated sample shows the lowest μ among the three samples. The μ - T curve is not monotonic with a peak value of 31 cm 2 V −1 s −1 near 175 K. In contrast, μ monotonically increases for the MPS-treated samples on cooling. For T >100 K, μ ~ T − γ , where γ =0.72 and 0.64 for the DS-treated and TS-treated samples, respectively. For T <100 K, μ gradually saturates. At T =10 K, μ =320 cm 2 V −1 s −1 for the DS-treated sample, which is ~3 (22) times higher than the TS-treated (as-exfoliated) one. We stress that all the above-mentioned transport phenomena are reproducible among different samples. In Supplementary Fig. 12 , we show three additional sets of data for two-terminal devices. Although the mobility is lower than their corresponding four-terminal counterparts due to contact resistance, all the key transport properties, including MIT, scaling of mobility and conductivity, are qualitatively reproduced. Theoretical modelling of charge transport Although some theories have been proposed to explain the mobility of monolayer MoS 2 (refs 13 , 25 ), a more complete physical model remains to be developed to fully understand the charge transport. In particular, the model should establish the correlation between different transport regimes and the underlying microscopic scattering mechanisms, provide quantitative information about the samples, and project device performance based on realistic parameters. We start by calculating the mobility of monolayer MoS 2 . According to Matthiessen’s rule, the mobility for free carriers is expressed as where μ ph , μ CI and μ sr are mobility limited by phonons, CI and short-range scatterings, respectively (the calculation of each term is described in Methods). The incorporation of μ sr in our model is motivated by (i) TEM characterization that clearly shows the existence of short-range SV defects and (ii) the saturation of μ at low temperatures. We do not consider surface optical phonon scattering because the relatively high energy of the SiO 2 phonon modes makes them irrelevant to the low-field mobility phenomenon considered here [25] . The experimentally measured ‘effective’ field-effect mobility μ is not equal to the free-carrier mobility μ 0 , due to the presence of charge traps that limits the free carrier population. Recently, localized trap states within the bandgap have been observed in both exfoliated and CVD monolayer MoS 2 (refs 11 , 14 , 15 ). The impurity band from these trap states can introduce a mobility edge that strongly affects the charge transport [26] . In a simple picture [27] , transport is carried only by electrons in the extended states, that is, states above the mobility edge. This model, which does not account for the hopping between the localized states, has been very successful in modelling organic FETs [27] , [28] . Here we adopt the same model to extract important physical quantities such as the density of CI ( N i ) and trap states ( N tr ), while avoiding the complexity of dealing with the energy-dependent mobility and percolation effects in hopping transport [27] (the detailed calculation is described in Methods). The model is further justified by its excellent agreement with the experimental data over a broad range of temperature and carrier density. With the above model, we can now quantitatively understand the obtained experimental data. The solid lines in Fig. 3 are the best fitting results using the parameters listed in Table 1 . Remarkably, the scaling of mobility and conductivity with temperature and carrier density is well reproduced with a single set of parameters, suggesting that our model captures the essential physics. At low temperature and low carrier density, the calculated σ and μ are lower than experiments ( Fig. 3b,d–f ), presumably due to the omission of hopping transport in our model. Hence, the discrepancy is the largest for the as-exfoliated sample ( Fig. 3b,d ) as N tr is the highest. Table 1 The fitting parameters in our theoretical model for the three devices in Fig. 3 . Full size table The fitting parameters in Table 1 give considerable insights into the microscopic origin of impurities in MoS 2 . In all of our samples, μ is much lower than μ ph , indicating that phonon scattering does not play a significant role. Rather, the mobility is largely limited by CI and short-range scatterings. We notice that N i and μ sr are reduced by MPS treatment and are correlated for each sample, suggesting that CI partially shares the microscopic origin with short-range defects, most likely SV. CI also partially comes from the interface, as the DS-treated sample has much lower N i than TS-treated one. For the DS-treated sample, N i becomes comparable to that of SiO 2 substrate (0.24–2.7 × 10 11 cm −2 ) (refs 29 , 30 , 31 ), indicating that a large portion of SV is repaired. N tr is also partially due to SVs as it can be reduced by MPS treatment. However, N tr is an order of magnitude higher than N i for all the samples, pointing to contributions from additional sources. This could be due to the ambient species absorbed between MoS 2 and SiO 2 during exfoliation, which act as charge traps as in the case of graphene [29] , [31] , [32] . For the MPS-treated samples, the high-temperature mobility is limited by CI, leading to the usual T − γ scaling behaviour. [13] predicts γ ~1 for the range of carrier densities studied here. However, both short-range scattering (temperature independent) and thermal excitation from charge traps (which leads to the opposite trend since the density of electrons in the extended states n c increases with temperature) can decrease the effective γ as observed here. Therefore, one cannot reliably infer the scattering mechanism solely by analysing γ . When the charge traps become dominant (which usually happens at low temperature and low carrier density), the mobility even exhibits an insulating behaviour as commonly observed in backgated devices [2] , [11] , [12] and in the as-exfoliated sample here ( Fig. 3b ). The mobility increases with carrier density for all three samples from the combined effect of CI and charge traps ( Fig. 3c ). Below a threshold carrier density (equivalent to mobility edge), μ becomes negligible due to the localized nature of electrons in charge traps. The mobility edge is found to decrease with temperature ( Supplementary Fig. 13 ) because of the thermal excitation of electrons to the extended states. At T =80 K, the threshold density is about 2 × 10 12 , 3 × 10 12 and 5 × 10 12 cm −2 for the DS-treated, TS-treated and as-exfoliated samples, respectively ( Fig. 3c ). These values are on the same order of magnitude with N tr , further supporting the charge trap model. Finally, we can also understand MIT in the framework of charge traps. Strong electron–electron correlation in 2D electron gas has been proposed to explain the MIT in monolayer MoS 2 , which gives a universal threshold density n MIT ~10 13 cm −2 (ref. 2 ). In our experiments, however, n MIT is apparently dependent on sample quality ( Fig. 3 ). The MIT can be intuitively understood from equation (6) (Methods). When n < N tr , the density of conducting electrons in the extended states ( n c ) is exponentially dependent on temperature due to thermal activation, the temperature dependence of σ is dominated by n c , showing thermally activated insulating behaviour [2] , [11] , [12] , [14] . For even smaller n and T , transport is dominated by variable-range hopping because n c can be ignored [11] , [14] ( Fig. 4a ). When n > N tr , the Fermi level is above the mobility edge and n c is independent of temperature. Thus, the temperature dependence of σ is dominated by μ 0 , showing metallic behaviour. Therefore, MIT occurs when n ≈ N tr . Using the trap and CI parameters of the DS-treated sample in Table 1 , we numerically calculated σ(n,T) (equation (6)) and obtained the n and T of each critical point as in Fig. 3f . 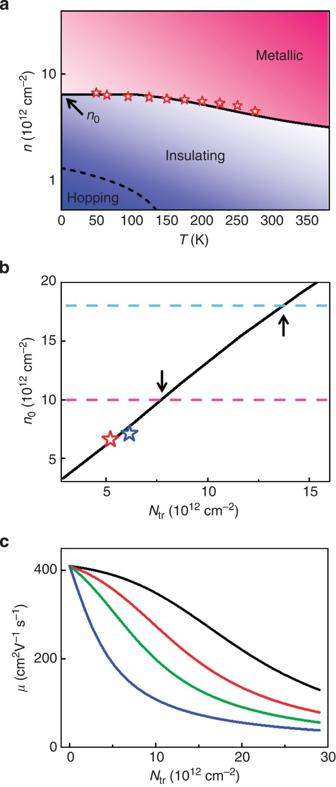Figure 4: Theory of charge transport in MoS2. (a) Phase diagram of charge transport in monolayer MoS2. The solid black line plots the calculated MIT critical points (using the parameters of DS-treated sample inTable 1) that separate the metallic and insulating regimes. The red symbols are experimental MIT points extracted fromFig. 3f. The lower left corner of the phase diagram illustrates the hopping transport regime (not calculated). (b) The solid black line is the calculatedn0as a function ofNtrusing the parameters of DS-treated sample inTable 1. The MIT curves under differentNtrare plotted inSupplementary Fig. 14. The blue and red symbols are experimental points from the TS-treated and DS-treated samples inFig. 3, respectively. We use the highestnthat exhibits MIT asn0. The horizontal dashed lines are MIT critical density estimated from refs2,9, respectively. The intersections with the solid line represent the estimate ofNtrin their devices (black arrows). (c) Theoretical calculation ofμas a function ofNtratT=300 K without any CI or short-range scatterings (using the parameters of DS-treated sample inTable 1). From top to bottom,n=2.0, 1.2, 0.7 and 0.16 × 1013cm−2, respectively. The phonon-limited value of 410 cm2V−1s−1is recovered atNtr=0. Figure 4a shows the calculated transport phase diagram with metallic and insulating regions. Excellent agreement with experiment is achieved without any fitting parameters, showing the consistency of our model. From Fig. 4a , n MIT slowly increases with decreasing temperature and converges to n 0 at T =0K. When n > n 0 , metallic behaviour is always expected. When n < n 0 , MIT is always expected at finite temperature. Under realistic trap and CI parameters, n 0 is linearly proportional to, but slightly higher than N tr ( Fig. 4b ; Supplementary Fig. 14 ). Therefore, n 0 can be used as a rough estimate of N tr . After careful comparison with literature [2] , [9] , [14] , [33] , we find that the N tr of our MPS-treated samples is indeed the lowest ( Fig. 4b ), indicating the highest sample quality. Figure 4: Theory of charge transport in MoS 2 . ( a ) Phase diagram of charge transport in monolayer MoS 2 . The solid black line plots the calculated MIT critical points (using the parameters of DS-treated sample in Table 1 ) that separate the metallic and insulating regimes. The red symbols are experimental MIT points extracted from Fig. 3f . The lower left corner of the phase diagram illustrates the hopping transport regime (not calculated). ( b ) The solid black line is the calculated n 0 as a function of N tr using the parameters of DS-treated sample in Table 1 . The MIT curves under different N tr are plotted in Supplementary Fig. 14 . The blue and red symbols are experimental points from the TS-treated and DS-treated samples in Fig. 3 , respectively. We use the highest n that exhibits MIT as n 0 . The horizontal dashed lines are MIT critical density estimated from refs 2 , 9 , respectively. The intersections with the solid line represent the estimate of N tr in their devices (black arrows). ( c ) Theoretical calculation of μ as a function of N tr at T =300 K without any CI or short-range scatterings (using the parameters of DS-treated sample in Table 1 ). From top to bottom, n =2.0, 1.2, 0.7 and 0.16 × 10 13 cm −2 , respectively. The phonon-limited value of 410 cm 2 V −1 s −1 is recovered at N tr =0. Full size image From the above discussion, it is clear that the transport in current state-of-the-art monolayer MoS 2 samples is still limited by charge traps, CI and short-range defects. To reach the real potential of monolayer MoS 2 in high-performance devices, continuous improvement of sample and interface quality is still needed. In Fig. 4c , we project the room-temperature mobility as a function of N tr in the ideal case, that is, without CI and short-range scattering. The mobility at low carrier density is rapidly degraded by even a small N tr . At a modest n =7 × 10 12 cm −2 , N tr has to be lower than 8.8 × 10 11 cm −2 , which is ~6 times lower than our DS-treated device, to achieve mobility >400 cm 2 V −1 s −1 . In conclusion, we have shown that thiol chemistry is an effective approach to engineer the defects and interface in monolayer MoS 2 towards intrinsic charge transport. A physical model that includes charge traps and major scattering sources has been developed to comprehensively describe the charge transport in MoS 2 and to quantify the density of CI and charge traps in the samples. We believe that our model captures the essential charge transport physics for monolayer MoS 2 and can be readily extended to other 2D semiconductors [33] , [34] , [35] . Density functional theory calculations Density functional theory calculations were performed using the Vienna ab initio simulation package (VASP) [36] , [37] . Projector-augmented-wave [38] potentials were used to describe ion–electron interactions, and the exchange correlation potential was represented by the local density approximation [39] . We used the climbing-image nudged elastic band method to locate the minimum energy paths and the transition states [40] . The defective MoS 2 sheet was modelled by a 4 × 4 supercell of MoS 2 with a single SV. A k-point sampling of 5 × 5 × 1 was used for all the calculations. MoS 2 sample preparation and MPS treatment In this work, we exfoliated monolayer MoS 2 from natural bulk flakes (SPI Supplies). The as-exfoliated samples were directly exfoliated on 300 nm SiO 2 /Si substrate. Before device fabrication, the samples were annealed in a mixture of H 2 /Ar at 350 °C to remove organic residue. For the TS-treated samples, we first exfoliated monolayer MoS 2 on 300 nm SiO 2 /Si substrate, followed by annealing in a mixture of H 2 /Ar at 350 °C to remove organic residue. The sample was then dipped in a fresh solution of 1/15 (v/v) MPS/dichloromethane for 24 h in a dry glove box to grow MPS on MoS 2 . After growth, the sample was taken out, rinsed thoroughly with dichloromethane and isopropanol (IPA), and blown dry with N 2 . Finally, the sample was annealed in a mixture of H 2 /Ar at 350 °C for 20 min to finish the MPS treatment and remove the extra MPS on MoS 2 ( Supplementary Fig. 3 ). For DS-treated samples, the 300 nm SiO 2 /Si substrate was first subject to a 30-min UV/ozone treatment to enhance surface hydrophilicity. The substrate was then dipped in a 10% (v/v) MPS/dichloromethane solution for 12 h in a dry glove box to grow MPS SAM. After the SAM growth, the substrate was sonicated in dichloromethane followed by thorough rinsing with dichloromethane and IPA, and drying with N 2 ( Supplementary Fig. 3 ). We then exfoliated monolayer MoS 2 on the SAM-treated SiO 2 /Si substrate. After exfoliation, the sample was dipped in a fresh solution of 1/15 (v/v) MPS/dichloromethane for 24 h in a dry glove box to grow MPS on the top side of MoS 2 , followed by thorough rinsing. Finally, the sample was annealed in a mixture of H 2 /Ar at 350 °C for 20 min to finish the MPS treatment. Device fabrication and electrical measurement We used standard photolithography to pattern the electrodes of MoS 2 backgated FETs on 300 nm SiO 2 /Si substrates. Ti/Pd (20 nm/20 nm) was electron beam evaporated as the contact metal for source, drain and voltage probes, followed by lift-off. All devices were annealed at 350 °C in Ar to improve contacts. Electrical measurements were carried out by an Agilent B1500 semiconductor parameter analyser in a close-cycle cryogenic probe station with base pressure ~10 −5 Torr. Before electrical measurements, a vacuum annealing at base pressure was performed to remove adsorbates and improve device performances [41] . TEM characterizations To prepare TEM samples, monolayer MoS 2 was first exfoliated on 300nm SiO 2 /Si substrate. We then align-transferred the sample to a copper TEM grid by the PMMA-based transfer method described in ref. 11 . The high-resolution TEM images were recorded in an image aberration-corrected TEM (FEI Titan 80–300 at 80 kV) equipped with a charge-coupled device camera (GatanUltraScanTM 1000). The exposure time was 1 s. Before recording, we set the third-order spherical aberration in the range of 1–6 μm and then we recorded the images under slightly underfocused. To minimize irradiation damage and prevent new SVs generating during normal imaging [24] , we limited the total exposure time to <30 s and the current density to <10 6 e nm −2 s −1 . A band-pass filter to the Fast Fourier Transformation of the original images was applied to enhance the visibility of the defects. Theoretical modelling The phonon-limited mobility is numerically calculated according to ref. 7 : where the coefficients α 1 =2.625 × 10 5 cm 2 K V −1 s −1 and α 2 =6.297 × 10 6 cm 2 K V −1 s −1 satisfy the boundary condition that μ ph (300 K ) =410 cm 2 V −1 s −1 and that μ ph ( T ) is continuous at 100 K. The transition at 100 K is due to the different phonon modes that limit the mobility [7] . The CI-limited mobility is calculated by the model described in ref. 13 : where f(E) is the equilibrium Fermi-Dirac distribution function and Γ imp is the electron momentum relaxation rate given by where is the screened scattering potential for a single CI. The expression and derivation for can be found in ref. 13 . Physically speaking, includes the effect of temperature-dependent charge polarizability on the electron screening of the charged impurity, which dominates the temperature dependence of the mobility at low and room temperature. The expression also implies that μ CI is inversely proportional to N i . Hence, from the fitting of the μ CI to the total effective mobility data, we are able to quantify the N i within the MoS 2 . As an example, Supplementary Fig. 15 plots μ CI as a function of T under N i =10 12 cm −2 . The short-range scattering-limited mobility μ sr is a constant fitting parameter that does not depend on temperature or carrier density [8] . To model the effect of charge traps, we assume the charge traps are uniformly distributed within ΔE tr below the conduction band edge ( Supplementary Fig. 16 ). We only consider shallow traps as the density of deep traps is at least an order of magnitude lower [14] , and that deep traps do not affect mobility and conductivity [27] . The Fermi energy E F (n, T) is determined by where N 0 =(2 m *)/( π ℏ 2 )=3.8 × 10 14 eV −1 cm −2 is the density of states in the conduction band, and m *=0.45 m e is the conduction band effective mass [42] . The density of conducting electrons in the extended states is The conductivity is calculated by and the ‘effective’ mobility is given by How to cite this article: Yu, Z. et al. Towards intrinsic charge transport in monolayer molybdenum disulfide by defect and interface engineering. Nat. Commun. 5:5290 doi: 10.1038/ncomms6290 (2014).